Stable platinum nanoparticles on specific MgAl2O4spinel facets at high temperatures in oxidizing atmospheres The development of thermally stable, nanometer-sized precious metal-based catalysts remains a daunting challenge. Such materials, especially those based on the use of costly platinum metal, are essential and, to date, non-replaceable for a large number of industrially important catalytic processes. Here we report a well-defined cuboctahedral MgAl 2 O 4 spinel support material that is capable of stabilizing platinum particles in the range of 1–3 nm on its relatively abundant {111} facets during extremely severe aging at 800 °C in air for 1 week. The aged catalysts retain platinum dispersions of 15.9% with catalytic activities for methanol oxidation being ~80% of that of fresh ones, whereas a conventional Pt/γ-Al 2 O 3 catalyst is severely sintered and nearly inactive. We reveal the origin of the markedly superior ability of spinel {111} facets, resulting from strong interactions between spinel surface oxygens and epitaxial platinum {111} facets, inspiring the rational design of anti-sintering supported platinum group catalysts. Supported platinum catalysts exhibit superior catalytic activity and are not readily substituted for many industrially important catalytic processes. The characteristics of the supported noble metal nanoparticles, such as crystallite size, shape and exposing facets, are crucial to catalytic activity and selectivity [1] , [2] . As a straightforward example, nanosized Pt nanoparticles provide high surface-to-volume ratios that, in turn, optimize the availability of the catalytically active surface atoms [3] , an especially important consideration in view of the high cost of Pt. Unfortunately, Pt particles of such small sizes are often not stable under realistic reaction conditions on commonly used catalyst support materials, especially at temperatures of >600 °C and under oxidizing atmospheres [4] as a result of a number of possible processes. For example, at very high temperatures (typically >1,000 °C), Pt transport via gaseous PtO 2 is considerable and can even result in Pt loss from the catalysts [5] . At lower temperatures, depending on the interactions between the support material and Pt, two primary mechanisms ( Fig. 1 ) for the loss of small Pt particles are particle growth (‘sintering’ over Al 2 O 3 , SiO 2 , TiO 2 , ZrO 2 oxide supports) [6] or reaction with the support material (leading sometimes to the formation of MPtO x solid solutions, M=Mg, Ce) [7] , [8] . The reduction in the number of accessible small Pt particles on all of these supports induces a decrease in the amount of exposed metallic Pt atoms and always results in a dramatic loss in catalytic reactivity. To re-disperse the sintered Pt particles or regenerate inactive MPtO x species, inefficient and expensive oxy-chlorination and/or H 2 -reduction treatments are typically required [7] , [8] , [9] . In view of these issues, thermally stable Pt catalysts under oxidizing atmospheres are extremely desirable in the industry. 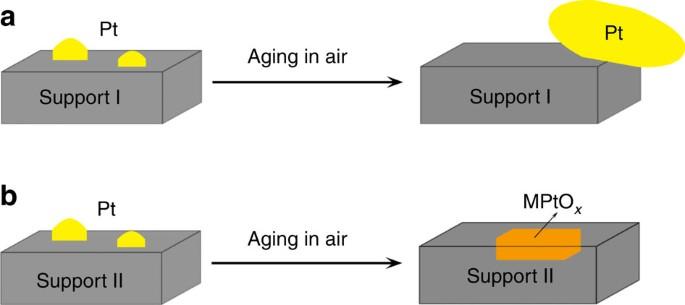Figure 1: Deactivation modes. Deactivation modes for small Pt particles on different supports during aging under oxidizing atmospheres. (a) Pt sintering over ’Type l‘ (Al2O3, SiO2...) support surface. (b) Solid-state reactions of supported Pt with ’Type ll‘ support materials (CeO2, MgO...), leading to dissolution of Pt into the bulk support. Figure 1: Deactivation modes. Deactivation modes for small Pt particles on different supports during aging under oxidizing atmospheres. ( a ) Pt sintering over ’Type l‘ (Al 2 O 3 , SiO 2 ...) support surface. ( b ) Solid-state reactions of supported Pt with ’Type ll‘ support materials (CeO 2 , MgO...), leading to dissolution of Pt into the bulk support. Full size image Attempts to stabilize small Pt metal nanoparticles are frequently reported in the literature. For the materials with weak interaction with Pt, one popular strategy is to form barriers to inhibit the migration of Pt particles by constructing specific support structures such as nanoparticles, films, shells and pores [10] , [11] , [12] , [13] , [14] , [15] . With this approach, only comparatively large (~10–15 nm) Pt particles have been successfully encapsulated in a porous silica shell and demonstrate enhanced stability after severe thermal treatments [10] . To utilize strong interactions between some oxide materials and Pt, these oxides are sometimes used as promoters by being dispersed along with Pt on the primary catalyst support material [16] , [17] . These approaches indeed show some enhanced stabilization of small Pt metal particles, although the detailed mechanism of stability is not yet clear. In spite of these promising recent developments, to date there are still no reliable and commercially viable approaches to stabilizing nanometer-sized catalyst metal particles. The spinel phase of the mixed oxide, magnesium aluminate (MgAl 2 O 4 ), is thermally stable and may represent an improved material that combines useful properties of other catalyst support materials, including expectations of moderate interaction with Pt, as Mg and Al atoms are present as alternating layers at the atomic level. The use of MgAl 2 O 4 as a support material for metal catalysts is not common but sometimes is chosen when particularly harsh reaction conditions are encountered, for example, in the reforming of methane [18] , [19] . In these cases, the stability of the MgAl 2 O 4 support material itself and its lack of acidity are essential properties [20] . MgAl 2 O 4 has occasionally been used as support material for platinum catalysts [21] , [22] , with the ability of MgAl 2 O 4 to stabilize small Pt nanoparticles reported to be ‘remarkable’ [21] . However, the reaction and aging conditions used in this prior study were relatively modest in severity with testing limited to 600 °C in oxidizing and reducing atmospheres. Furthermore, the origins of this enhanced stability remain unclear although the authors suggest the importance of strong interactions between PtO x species and surface oxide ions [21] . Spinel MgAl 2 O 4 has a face-centered cubic (FCC) Bravais lattice with a space group Fdm where all of the O 2− anions are arranged at slightly deformed FCC positions in the bulk [23] . Within the FCC-like oxygen sublattice, the Mg 2+ and Al 3+ atoms occupy 1/8 tetrahedral positions and 1/2 octahedral positions, respectively. MgAl 2 O 4 is usually prepared by solid state reactions between magnesium and aluminium oxides or their hydroxides, where inhomogeneities in local composition, structure and morphology are common [24] , significantly complicating the identification of surface structure. As such, addressing the origin of Pt metal stability on these materials will not be simple. In this paper, we report the preparation of a pure MgAl 2 O 4 spinel material having primary cuboctahedral shape with dominant {100} and {111} facets, and its use as a catalyst support for Pt. Significantly, the well-defined MgAl 2 O 4 spinel composition and structure in these materials enables the study of interactions between Pt nanoparticles and specific surface facets. We also report the very surprising thermal stability of Pt nanoparticles on these well-defined MgAl 2 O 4 support materials during highly severe thermal aging in oxidizing atmospheres. This stability in Pt nanoparticle size is also evident in the rates of methanol oxidation at low temperature after varying aging treatments. To rationalize this stability, we present high-resolution transmission electron microscopy (HR-TEM) images that provide clear evidence for the presence of small Pt nanoparticles (1–3 nm) that are epitaxially oriented with the MgAl 2 O 4 spinel {111} facets even after the most severe thermal aging at 800 °C in air for 1 week. We also describe density functional theory (DFT) calculations that reveal the likely origin of unusual stability on the preferred surfaces. Catalyst synthesis and treatment Magnesium aluminate spinel supports were prepared by hydrolysis of aluminium isopropoxide with magnesium nitrate hexahydrate in ethanol as described in the Methods section. Pt catalysts supported on the spinel and traditional γ-Al 2 O 3 (for comparison) materials were prepared by incipient wetness impregnation. The platinum loading was 1 wt%, which resulted in nearly identical Pt surface coverages for these catalysts (1Pt/MgAl 2 O 4 and 1Pt/γ-Al 2 O 3 ). Following drying and calcination at 500 °C for 5 h, the ‘fresh’ samples were then reduced in 5% H 2 /He at 800 °C for 2 h. After this high-temperature reduction, residual chloride on the samples was below the XPS detection limit (0.1% surface atomic ratio). Thus, the influence of Cl − on reactivity and Pt stability [14] can be neglected. As severe sintering of Pt usually occurs during long-term high-temperature treatment in oxidizing atmospheres, the reduced samples were subsequently aged in ambient air at 800 °C for both 1 day (24 h, ‘1D’) and 1 week (168 h, ‘1 W’), respectively. These aged samples were also subsequently reduced in 5% H 2 /He at 800 °C for 2 h. We denote the calcining treatment as ‘O’ and that of H 2 reduction as ‘R’. Thus, these samples are designated with a suffix of ‘-FO’ and ‘-FR’ (that is, fresh-oxidized and fresh-reduced, respectively), or ‘-1DO’ and ‘-1DR’, or ‘-1WO’ and ‘-1WR’, respectively (the protocols for preparing and thermally treating the Pt/MgAl 2 O 4 and Pt/γ-Al 2 O 3 catalysts as well as the nomenclature used here are summarized in Supplementary Fig. S1 ). These catalysts were characterized before and after aging by a variety of techniques including HR-TEM and X-ray diffraction (XRD), and assessed for catalytic performance using a model methanol oxidation reaction. Thermal stability Freshly prepared 1Pt/MgAl 2 O 4 -FR shows a high Pt dispersion (via H 2 chemisorption) of 36.3% with small particle sizes of 1–3 nm as evidenced by TEM ( Fig. 2a ) and the fact that Pt is not detected in XRD ( Fig. 3 ), a technique with a detection limit of ~3 nm. After aging, the Pt dispersions decreased modestly to 29.1 and 15.9% for 1Pt/MgAl 2 O 4 -1DR and 1Pt/MgAl 2 O 4 -1WR, respectively ( Fig. 4a ). Most of the Pt nanoparticles are in the 1–3 nm range, but a few large Pt particles of ~20 or 50 nm are also revealed in the TEM images for 1Pt/MgAl 2 O 4 -1DR ( Fig. 2b ) and 1Pt/MgAl 2 O 4 -1WR ( Fig. 2c ). These observations are consistent with XRD results ( Fig. 3 ), although XRD will be primarily sensitive to the largest particles and thus somewhat overestimate the average size of the large Pt particles with a Scherrer equation analysis ( Supplementary Table S1 ) [25] . However, by using a quantitative multi-component Rietveld analysis of the powder diffraction patterns [26] , [27] we can provide a useful estimate of the relative number of small and large Pt particles by assuming we have the approximate bimodal distribution of sizes observed in the TEM data. In this way, we estimate that ~10 and 40% of Pt forms large particles in 1Pt/MgAl 2 O 4 -1DR and -1WR, respectively ( Supplementary Table S1 ), values that are in line with the loss in Pt dispersions determined with H 2 chemisorption measurements. Thus, taken together the results from these three techniques provide a consistent picture of a bimodal Pt size distribution after extended 1-week aging, with Pt particles in size ranges of ~1–3 and ~20–50 nm. Here, we also note that the inset to Fig. 2b shows a large Pt particle of ~25 nm with a considerable number of small (~1–3 nm) Pt particles attached, indicating that large Pt particles may grow via coalescence of small ones that detach from the support as discussed in more detail below. 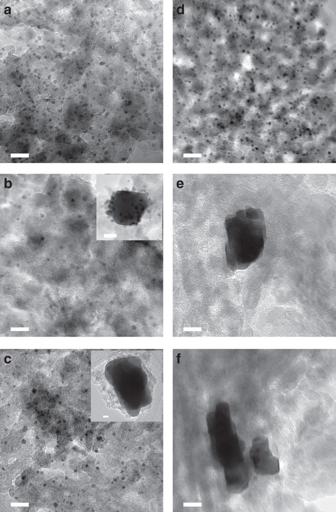Figure 2: TEM analysis. TEM images for 1Pt/MgAl2O4: -FR (a), -1DR (b) and -1WR (c); and for 1Pt/γ-Al2O3: -FR (d), -1DR (e) and -1WR (f) samples. Scale bars are all 10 nm. Figure 2: TEM analysis. TEM images for 1Pt/MgAl 2 O 4 : -FR ( a ), -1DR ( b ) and -1WR ( c ); and for 1Pt/γ-Al 2 O 3 : -FR ( d ), -1DR ( e ) and -1WR ( f ) samples. Scale bars are all 10 nm. 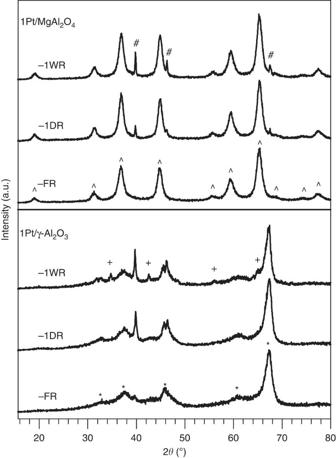Figure 3: XRD analysis. XRD patterns for 1Pt/MgAl2O4and 1Pt/γ-Al2O3samples. The ‘^’, ‘*’, and ‘#’ and ‘+’ marks indicate the diffraction peaks for MgAl2O4spinel, γ-Al2O3, and metallic Pt, and α-Al2O3, respectively. Full size image Figure 3: XRD analysis. XRD patterns for 1Pt/MgAl 2 O 4 and 1Pt/γ-Al 2 O 3 samples. The ‘^’, ‘*’, and ‘ # ’ and ‘ + ’ marks indicate the diffraction peaks for MgAl 2 O 4 spinel, γ-Al 2 O 3 , and metallic Pt, and α-Al 2 O 3 , respectively. 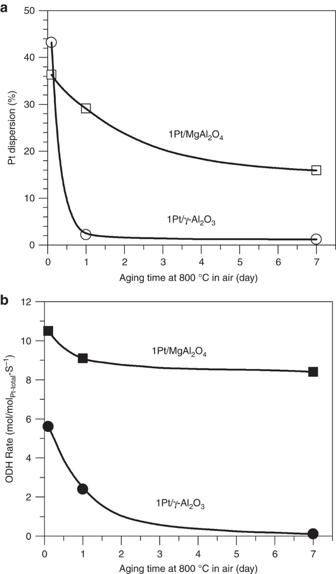Figure 4: Pt dispersion and reactivity. Pt dispersions obtained from H2chemisorption measurements (a), and steady-state methanol ODH rates normalized to the total amount of Pt (b) for the 1Pt/MgAl2O4and 1Pt/γ-Al2O3samples with varying aging time. Full size image Figure 4: Pt dispersion and reactivity. Pt dispersions obtained from H 2 chemisorption measurements ( a ), and steady-state methanol ODH rates normalized to the total amount of Pt ( b ) for the 1Pt/MgAl 2 O 4 and 1Pt/γ-Al 2 O 3 samples with varying aging time. Full size image For a conventional Pt/γ-Al 2 O 3 sample, the Pt dispersion of freshly prepared 1Pt/γ-Al 2 O 3 -FR was 43.2% and sharply decreased to 2.2% and then to 1.2% for 1Pt/γ-Al 2 O 3 -1DR and 1Pt/γ-Al 2 O 3 -1WR, respectively ( Fig. 4a ). Small Pt particles (<3 nm) present for 1Pt/γ-Al 2 O 3 -FR disappeared completely for 1Pt/γ-Al 2 O 3 -1DR and 1Pt/γ-Al 2 O 3 -1WR samples ( Fig. 2b,d,f ); meanwhile, increasingly larger Pt particles appeared, thus displaying a typical sintering process. It is important to note that Pt was already sintered to a significant extent for the 1Pt/γ-Al 2 O 3 -1DR sample. In particular, this sample showed essentially no evidence in XRD ( Fig. 3 ) for the transformation of γ-Al 2 O 3 to other phases, a process sometimes regarded as a cause for Pt sintering in these type of supported catalysts. These results, summarized in Supplementary Table S1 , demonstrate that nano-sized Pt particles on the spinel MgAl 2 O 4 support are significantly more stable in the severe aging conditions used here. Catalytic reactivity To compare the reactivity and Pt utilization of the variously treated catalysts studied here, we report Pt mass-specific rates of methanol oxidative dehydrogenation (ODH), a widely used surface probe reaction [28] , [29] , [30] . Note that the reaction of the bare MgAl 2 O 4 support is negligible as shown in Supplementary Fig. S2 . As shown in Fig. 4b , the steady-state mass-specific ODH rates for 1Pt/MgAl 2 O 4 -FR, -1DR and -1WR decrease slightly from 10.5 to 9.1 and then to 8.4 mol/mol Pt-total -S −1 (these rates are also summarized in Supplementary Table S2 ). That is, the catalytic activities of the severely aged catalysts, 1Pt/MgAl 2 O 4 -1DR and -1WR, were at least 80% of that for the freshly prepared 1Pt/MgAl 2 O 4 -FR catalyst. This behaviour is in significant contrast to methanol ODH activities measured for the fresh and aged γ-Al 2 O 3 -supported catalysts. In particular, the steady-state ODH rates for 1Pt/γ-Al 2 O 3 -FR, -1DR and -1WR decreased dramatically from 5.6 to 2.4, and then to 0.1 mol/mol Pt-total -S −1 , indicating significant loss of catalytic activity entirely consistent with the extent of Pt sintering observed with TEM and XRD. Turnover frequencies (TOFs) are also reported in Supplementary Table S2 by normalizing the ODH rates to the number of surface Pt atoms measured with H 2 chemisorption. TOFs generally increase with aging for both catalysts indicating that more thermodynamically stable Pt surfaces may be somewhat more active [31] . Note, however, that TOFs for aged Al 2 O 3 -supported catalysts are less reliable due to uncertainties in the H 2 chemisorption measurements for materials with significant Pt sintering. Structure of Pt/MgAl 2 O 4 The markedly superior thermal stability and catalytic activity of Pt/MgAl 2 O 4 catalysts indicates that their structures are unique. As shown in Fig. 5a , the spinel crystallites in 1Pt/MgAl 2 O 4 -FR show tetragonal and hexagonal or pseudo-hexagonal projections. Using geometry analysis, these projections are most likely from cuboctahedrons: a tetragon could be a projection of a cuboctahedron along the [001] direction, whereas a long or regular hexagon might be projections along [110] or [111] directions, respectively ( Fig. 5b ). Pseudo-hexagonal and even irregular projections can also appear cuboctahedrons are viewed in other directions. For example, Supplementary Fig. S3 demonstrates that a typical hexagonal projection will appear as irregular projections on tilting the sample from top view to side view. Irregular projection may also lead to truncated-cubes if the cuboctahedron is not well-developed. For a perfect cuboctahedron, the surface areas of {100} and {111} are nearly identical. The transformation of cubic spinel to truncated-cube and to cuboctahedron creates more {111} surface at the expense of {100}, and results in more thermodynamically favourable shapes [32] . In Fig. 5a , Pt particles are also evident yet are sometimes too small for their shapes to be determined. For the somewhat larger Pt particles in the image, hexagonal shapes are evident indicating some geometrical relationship to the shapes of the MgAl 2 O 4 particles. 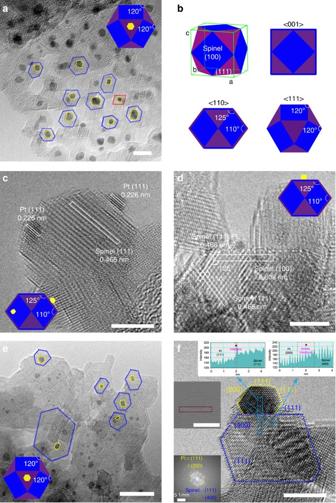Figure 5: HRTEM analysis. HRTEM images for Pt/MgAl2O4-FR (a,c, andd) and Pt/MgAl2O4-1WR (e,f). Scale bars are all 5 nm. Also shown is an ideal cuboctahedron structure and its 2-D projections along [001], [110] and [111] directions (b). In (f), the epitaxial relationship between Pt and spinel support is documented by the continuity of (400)MgAl2O4and (200)Ptlattice fringes across the atomically flat interface. This figure also includes an inset that shows lattice fringe intensity profile across the two structures. The FFT analysis in another inset depicts diffraction spots from both structures having perfect lattice matching. The diffraction spots are indexed and show matching of (400)MgAl2O4/(200)Ptand (222)MgAl2O4/(111)Pt. Finally, another inset shows a band-pass filter image recreated from the FFT with spatial frequencies from 3 nm−1to 6.8 nm−1and clearly showing details of the epitaxial interface. Figure 5: HRTEM analysis. HRTEM images for Pt/MgAl 2 O 4 -FR ( a , c , and d ) and Pt/MgAl 2 O 4 -1WR ( e , f ). Scale bars are all 5 nm. Also shown is an ideal cuboctahedron structure and its 2-D projections along [001], [110] and [111] directions ( b ). In ( f ), the epitaxial relationship between Pt and spinel support is documented by the continuity of (400) MgAl2O4 and (200) Pt lattice fringes across the atomically flat interface. This figure also includes an inset that shows lattice fringe intensity profile across the two structures. The FFT analysis in another inset depicts diffraction spots from both structures having perfect lattice matching. The diffraction spots are indexed and show matching of (400) MgAl2O4 /(200) Pt and (222) MgAl2O4 /(111) Pt . Finally, another inset shows a band-pass filter image recreated from the FFT with spatial frequencies from 3 nm −1 to 6.8 nm −1 and clearly showing details of the epitaxial interface. Full size image Besides having a similar shape as the MgAl 2 O 4 particles, Fig. 5a demonstrates that Pt particles are very often located near the centres of the MgAl 2 O 4 particles. In this regard, it is important to note that the centres for tetragon and regular hexagon projections give rise to square (100) and triangle (111) facets, respectively, whereas that for the long hexagon is a corner of the cuboctahedron. Furthermore, as superimposed in Fig. 5a , many of the spinel particles with a hexagonal or pseudo-hexagonal shape are the ones with a Pt particle on the centre. These are most likely <111> oriented spinel particles with a {111} facet at the centre. Especially interesting is that most of the Pt particles located at the centre of the spinel particles have hexagonal or pseudo-hexagonal shapes, suggesting that a commonly realized interface for the Pt particles and the spinel particles is the {111} surface. Although the low-magnification TEM image in Fig. 5a suggests that Pt particles are frequently located on the (111) spinel surfaces, an HRTEM study indicates that Pt particles can be observed on both (111) and (100) facets for the fresh catalysts (that is, prior to exposure to severe aging conditions), for example, Fig. 5c is an HRTEM image observed along [110] with two Pt particles on one MgAl 2 O 4 spinel crystallite. Such a plane-view HRTEM image enables a more-specific view of the interacting surfaces: one Pt particle located on a spinel (111) facet and the other is on a spinel (100) facet as illustrated in the figure’s insert (‘inset’ is used elsewhere). Figure 5d shows a Pt particle on spinel (100). Thus, Pt particles are observed on both {100} and {111} facets for the 1Pt/MgAl 2 O 4 -FR sample, displaying somewhat random occupation for Pt after initial dispersing. For the 1Pt/MgAl 2 O 4 -1WR sample, although there is modest coalescence and surface-area loss of the support appeared after the long term aging, Fig. 5e demonstrates that hexagonal spinel particles with a Pt near the centre clearly dominates for the observed Pt-containing particles. Tetragonal-shaped spinel particles with a Pt on the centre are very rare, if present at all, for several observed specimens. Figure 5f shows a high-resolution image of a small Pt crystallite located on a spinel (111) surface, indicating that this is the stable structure for small Pt particles on spinel supports surviving even very severe oxidative aging. Importantly, the high-resolution image in Fig. 5f displays a presence of continuous lattice fringes across the Pt particle and spinel support, documenting that the structures have an epitaxial relationship on the atomically flat (111) interface. The epitaxial relationship and the necessary lattice matching are more evident from an FFT analysis that depicts diffraction spots from both structures. The diffraction spots are indexed and show matching of the following lattice vectors: (400) MgAl2O4 /(200) Pt and (222) MgAl2O4 /(111) Pt . Additional HRTEM images also show small Pt epitaxially attaching on spinel (111) surfaces ( Supplementary Fig. S4 ). Some clear HRTEM images allow us to carry out Wulff–Kaichew constructions [33] ( Supplementary Fig. S5 ). In this way, the adhesion energy between Pt(111) and MgAl 2 O 4 (111) is estimated to be about half of the surface energy of Pt(111), showing very strong interaction [34] . Considering also the drop in Pt dispersion by half, and the essentially equal distribution of {111} and {100} surfaces, the structure of thermally stable Pt particles on spinel can be concluded to be those that attach to the spinel {111} facets. DFT calculations The relative thermal stability of Pt particles on spinel (111) and (100) surfaces was also theoretically simulated. Spinel MgAl 2 O 4 has a FCC Bravais lattice with a space group Fdm where the Mg 2+ and Al 3+ atoms occupy 1/8 tetrahedral positions and 1/2 octahedral positions of the FCC-like oxygen sublattice, respectively [23] . The stacking sequence for (100) is (-O-O-)\(-Al-)\(-O-O-)\(-Mg-) and that for (111) is (-O-O-O-)\(-O-)\(-Al-)\(-O-)\(-O-O-O-)\(-Mg-)\(-Al-)\(-Mg-). Previous theoretical calculations [35] , [36] have indicated that the O\(Mg-Al-Mg)-terminated MgAl 2 O 4 (111) surface and the Mg\O-terminated MgAl 2 O 4 (100) surface are the most stable surfaces with the lowest surface energies for each surface orientation even considering some concentration of Mg-Al antisites as reported for MgAl 2 O 4 (100) [37] . Considering that the spinel support has experienced long-term high-temperature calcination before use, these two surface slabs were therefore chosen as the representative structures for the spinel support on which the Pt particles deposit. To get a stoichiometric O\(Mg-Al-Mg)-terminated MgAl 2 O 4 (111) surface, half of the surface oxygens must be removed from a cleaved oxygen layer ( Supplementary Fig. S7 a,b). As Pt metal also has an FCC lattice, Pt atoms can first occupy the positions of the removed oxygen atoms and then stack in a FCC pattern as shown in Fig. 6a (top three layers in blue). This initial structure was annealed at 800 °C for 10 ps and the result is shown in Fig. 6b . The interfacial layer containing both oxygen and Pt atoms separated into two layers: an oxygen sub-layer and Pt upper layer with an average separation of 2.16 Å. This value is very close to the distance between two oxygen layers in bulk spinel (2.22 Å) or two Pt layers in bulk Pt (2.26 Å), indicating a strong interaction between interfacial oxygen and Pt and a good lattice match. To break the Pt-O bond in the aged catalyst model requires 1.37 eV for each interfacial Pt atom (averaged). 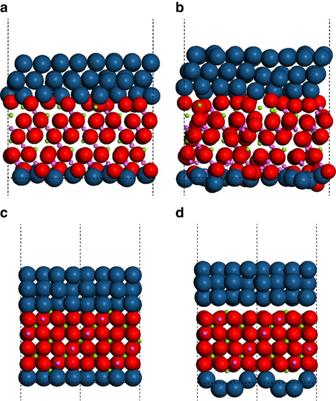Figure 6: DFT calculations. Initial structure of Pt atoms deposited on the O-terminated MgAl2O4(111) surface slab (a) and that at 800 °C (b). Initial structure of Pt atoms deposited on the Mg terminated MgAl2O4(100) surface (c) and that at 800 °C (d). The magnesium atoms are in green, the aluminium atoms in magenta, the oxygen atoms in red, and the Pt atoms are in blue. Figure 6: DFT calculations. Initial structure of Pt atoms deposited on the O-terminated MgAl 2 O 4 (111) surface slab ( a ) and that at 800 °C ( b ). Initial structure of Pt atoms deposited on the Mg terminated MgAl 2 O 4 (100) surface ( c ) and that at 800 °C ( d ). The magnesium atoms are in green, the aluminium atoms in magenta, the oxygen atoms in red, and the Pt atoms are in blue. Full size image For the Mg\O-terminated MgAl 2 O 4 (100) surface, half of the surface Mg atoms are removed to obtain stoichiometry of MgAl 2 O 4 . Pt atoms were then stacked on the surface in an FCC pattern as shown in Fig. 6c (top three blue layers). After annealing at 800 °C for 10 ps, the Pt layers moved entirely away from the spinel (100) surface with a distance between the bottom Pt layer and the spinel surface oxygens of 3.50 Å ( Fig. 6d ), clearly showing a detachment of Pt particles from the (100) surface. This simulation result is in line with the experimental observations, showing the importance of surface termination and lattice structure. As a further check on the effect of support surface structure on Pt stability, the simulations also included a single Pt layer below the MgAl 2 O 4 support ( Fig. 6 ). In this way, Pt is only able to interact with the support or with other Pt atoms in a 2D rather than 3D layer. Even in this case, the results again demonstrate the positive influence of lattice matching to the (111) surface in stabilizing the Pt monolayer. γ-Al 2 O 3 also belongs to the cubic system ( ). The commercial γ-Al 2 O 3 support used in this work has platelet-like shapes ( Supplementary Fig. S6 ), where the (110) and (100) surfaces are expected to be ~70–80% and 16–30%, respectively [38] . The γ-Al 2 O 3 (111), which is most promising for stabilizing Pt via lattice-matched interactions as indicated by similar calculations to the ones just described for MgAl 2 O 4 , is, at most, only a minor surface phase. As it offers the best chance for stabilizing Pt, in the Supplementary Fig. S7c,d , we show the simulated thermal stability of Pt on a γ-Al 2 O 3 (111) surface. Even in this case, the Pt layers move away from the γ-Al 2 O 3 (111) surface to an average distance of 3.7 Å after annealing at 800 °C for 10 ps ( Supplementary Fig. S7d ). However, to completely detach the Pt layers from the alumina support surface, only ~0.28 eV is required for each interfacial Pt atom. Thus, these simulations are in line with the rather poor thermal stability of the γ-Al 2 O 3 -supported Pt catalysts. Pt supported on other MgAl 2 O 4 spinel materials We have also studied commercially available spinel materials that typically have large particle sizes and low surface areas. The Pt dispersions and stability are very poor ( Supplementary Table S3 ). We also used spinel materials that were prepared by conventional co-precipitation methods. These latter catalyst supports have small particle sizes and high surface areas as well as similar dominant cuboctahedral shapes, but varying amounts of MgO and/or γ-Al 2 O 3 impurity phases ( Supplementary Fig. S8 ). In this case, as with the model spinel materials discussed above, Pt was highly dispersed and well stabilized, albeit somewhat poorer in both respects compared with the model catalyst supports ( Supplementary Table S3 ). Thus, somewhat lower percentages of {111} facets and/or Pt present on impurity γ-Al 2 O 3 and MgO phases may explain why varied results for Pt dispersions have been reported in past studies that used MgAl 2 O 4 spinel of other morphologies as Pt supports [21] , [22] . In this work, supported Pt catalysts with remarkable thermal stability were successfully prepared by taking advantage of the specific surface structure of MgAl 2 O 4 spinel supports via simple wetness impregnation methods, and the catalyst structures are presented in detail. Primary particles of the spinel support used here have a cuboctahedral shape that expose {100} and {111} facets. The well-defined morphology of these spinel support materials allows us to clearly demonstrate that small Pt particles (1–3 nm) on the small {111} spinel surfaces can survive severe aging, leading to the maintenance of high Pt dispersions, while those on {100} surfaces are sintered. Theoretical simulations reveal that O\(Mg-Al-Mg)-terminated spinel (111) surfaces favour the epitaxial growth of Pt in a lattice-matching manner. In the MgAl 2 O 4 spinel supports with a cuboctahedron shape, six {100} facets are isolated by eight {111} facets and the {100} and {111} intersecting plane angles are ~125°. The O\(Mg-Al-Mg)-termination of spinel (111) attracts Pt(111), whereas the Mg\O-termination of spinel {100} repels Pt(100). The large particles are formed via a sintering process ( Fig. 2b inset) and the source of Pt particles for coalescing seems to be those initially on spinel {100} surfaces. In view of the HRTEM results, the small particles on {111} facets did not appear to grow in size during aging, perhaps due to the small chance that the unstable small particles on {100} cross over the intersecting edge. The small dimensions of exposed {111} facets therefore limit the sizes of attached Pt particles, contributing to the prevention of Pt sintering and thus formation of large Pt particles. The Pt mass-specific catalytic reactivity of the aged spinel-supported catalysts, as probed by methanol ODH, retained 80% of that on the fresh one. This behaviour is in significant contrast to that observed for Pt catalysts on the more commonly used γ-Al 2 O 3 support material, where very low Pt dispersions and correspondingly low rates of reaction are observed after similar aging treatments. In view of the comparative catalyst characterization and performance measurements reported here, we conclude that enhancing the quantity of spinel {111} facets in a magnesium aluminate support materials may be a promising way to improve stability of Pt particles towards sintering, thus providing important information for the rational design of anti-sintering-supported platinum group catalysts. Synthesis and calcination of catalysts Magnesium aluminate spinel supports were prepared by hydrolysis of aluminium isopropoxide with magnesium nitrate hexahydrate in ethanol according to equation 1. Stoichiometric quantities of aluminium isopropoxide (98+%, Alfa Aesar) (0.1 mol) and magnesium nitrate hexahydrate (98%, Alfa Aesar) (0.05 mol) were mixed in 300 ml denatured ethanol in a 1,000 ml Pyrex bottle. The bottle was sealed and then put on a heating plate with magnetic stirring. After stirring for 1 h, the plate was heated to 150 °C and held there for 12 h. Then, the ethanol was evaporated and the resultant gel was dried at 90 °C overnight. Finally, the dried powders were calcined in ambient air at 800 °C for 12 h with a heating rate of 5 °C min −1 , resulting in the formation of MgAl 2 O 4 support materials with pure spinel crystal phase. Supported Pt catalysts were prepared by incipient wetness impregnation of MgAl 2 O 4 spinel and γ-Al 2 O 3 (Condea, 150 m 2 g −1 ) materials using aqueous solutions of PtCl 4 (99.9%, Alfa Aesar) at room temperature for 20 h. The platinum loading was 1 wt %. Impregnated samples were dried at 110 °C in ambient air overnight and then treated according to Supplementary Fig. S1 . They were first calcined at 500 °C for 5 h and then were reduced in 5% H 2 /He at 800 °C for 2 h. As severe sintering of Pt usually occurs during long-term high-temperature treatment in oxidizing atmospheres, the reduced samples were subsequently aged in ambient air at 800 °C for both 1 day (24 h, ‘1D’) and 1 week (168 h, ‘1 W’), respectively. The aged samples were also reduced in 5% H 2 /He at 800 °C for 2 h. We denote the calcining treatment of as ‘O’ and that of H 2 reduction as ‘R’. Thus, these samples are designated with a suffix of ‘-FO’ and ‘-FR’, or ‘-1DO’ and ‘-1DR’, or ‘-1WO’ and ‘-1WR’, respectively. Supplementary Figure S1 summarizes the protocol for preparing and thermally treating the Pt/MgAl 2 O 4 and Pt/γ-Al 2 O 3 catalysts as well as the nomenclature used here. For comparison, a commercial MgAl 2 O 4 material (99%, Alfa Aesar, denoted as MgAl 2 O 4 -a) and conventionally prepared MgAl 2 O 4 materials were also used as supports to prepare Pt catalysts. For the latter, stoichiometric quantities of Al(NO 3 ) 3 ·9H 2 O (98%, Alfa Aesar) (0.1 mol) and Mg(NO 3 ) 2 ·6H 2 O (0.05 mol) were dissolved in 300 ml distilled water. An aqueous solution of ammonia was dropped into the solution under stirring until the final pH value was ~9.5. The precipitate was continuously stirred for 12 h and then treated in two ways. One is to separate the precipitate by centrifugation and the other is to obtain the precipitate by evaporating water. Finally, the powders were calcined in ambient air at 800 °C for 12 h with a heating rate of 5 °C min −1 . The resultant materials are denoted as MgAl 2 O 4 -b and MgAl 2 O 4 -c for the centrifuged and evaporated samples, respectively. One difference for these latter two materials is that they contain different amounts of an MgO impurity phase ( Supplementary Fig. S8 ). Supported Pt catalysts on MgAl 2 O 4 -a, -b and -c were prepared and then thermally treated in the same way as described above for the model spinel materials. Catalyst characterization Surface areas were measured on a QuantaChrome Autosorb-6 using N 2 adsorption isotherms and BET analysis methods. All of the samples were degassed under vacuum at 150 °C for 4 h before the adsorption measurements. TEM was used to analyse the size and the morphology of the Pt particles. Conventional TEM analysis was performed with JEOL JEM 2010 operated at 200 keV with a specified point-to-point resolution of 0.194 nm. For more detailed work, high-resolution imaging was performed with aberration-corrected (image-corrected) FEI Titan 80–300 operated at 300 kV. The aberration correction enables sub-Angstrom resolution in phase-contrast imaging mode. TEM specimens were prepared by depositing a suspension of the powdered sample on a lacey carbon-coated copper grid. XRD patterns were measured on a Philips PW3040/00 X’Pert MPD system equipped with a Cu source ( λ =1.5406 A). Data analysis was accomplished using JADE (Materials Data, Inc., Livermore, CA, USA) as well as the Powder Diffraction File database (2003 Release, International Center for Diffraction Data, Newtown Square, PA, USA). Crystallite size and quantitative phase analysis were performed using Scherrer equation [25] , [39] and Rietveld method [26] , [27] , respectively. Pt dispersions were obtained by hydrogen pulse chemisorption using a thermal conductivity detector on a GC-7890 A at 50 °C. Before the chemisorption, the sample was heated to 800 °C for 0.5 h under 2% H 2 /N 2 and switched to N 2 and held for 0.5 h, then cooled down to 50 °C in N 2 . Simulations All DFT calculations were carried out using a CP2K package [40] , [41] , [42] . GGA–PBE functional [43] and the pseudopotentials of Geodecker, Teter and Hutter [44] , [45] , [46] were used in the calculations, with a cutoff energy of 300 Ry. A BFGS algorithm with SCF convergence criteria of 1.0 × 10 –6 a.u. was used in geometry optimizations. To explore the stability of the deposited Pt atoms on the spinel MgAl 2 O 4 substrate at high temperatures, ab initio molecular dynamics implemented in the CP2K package was used to simulate the Pt atoms deposited MgAl 2 O 4 surfaces at 1,073 K. The standard simulated annealing procedure of the ab initio molecular dynamics simulation was applied. The {111} surface slab with the size (11.4353 Å × 19.8066 Å × 19.4490 Å) and the {100} surface slab with the size of (8.0860 Å × 8.0860 Å × 19.9134 Å) were used. Catalytic methanol oxidation measurements Methanol oxidation reactions were carried out at atmospheric pressure in a fixed-bed microreactor. Catalysts powders (~1 mg), diluted with SiC powder (3 g) to prevent temperature gradients, were held at the middle of a quartz reactor between two layers of quartz wool. A k -type thermocouple in a thin quartz tube was inserted into the catalyst bed to measure and control the temperature. The reactants were 4% (molar ratio) methanol in purified air, which was produced by flowing air through a saturator maintained at 50 °C and then through a condenser in cooling water at 1.2 °C. The flow rate was 200 SCCM min −1 and the reaction temperature was 80 °C, resulting in methanol conversions lower than 15%. The outlet of the reactor to a six-way gas sampling valve was heated at 150 °C to avoid condensation of the products. Reactants and products were analysed by an on-line gas chromatograph (Agilent 7890 A) equipped with a molecular sieve of 5 A and a HayeSep T packed columns, and a thermal conductivity detector. Selectivities are reported on a carbon basis as the percentage of the converted methanol appearing in a given product. Mass-specific rates and turn over frequencies (TOFs) for primary methanol ODH to HCHO are reported based on total Pt or surface Pt atoms, respectively, where formation of every HCHO, HCOOCH 3 and CO 2 molecule requires one oxidative methanol dehydrogenation event. How to cite this article: Li, W.-Z. et al. Stable platinum nanoparticles on specific MgAl 2 O 4 spinel facets at high temperatures in oxidizing atmospheres. Nat. Commun. 4:2481 doi: 10.1038/ncomms3481 (2013).